Genome-wide association study identifies three novel susceptibility loci for severeAcne vulgaris Acne vulgaris (acne) is a common inflammatory disorder of the cutaneous pilo-sebaceous unit. Here we perform a genome-wide association analysis in the United Kingdom, comparing severe cases of acne ( n =1,893) with controls ( n =5,132). In a second stage, we genotype putative-associated loci in a further 2,063 acne cases and 1,970 controls. We identify three genome-wide significant associations: 11q13.1 (rs478304, P combined =3.23 × 10 −11 , odds ratio (OR)=1.20), 5q11.2 (rs38055, P combined =4.58 × 10 −9 , OR=1.17) and 1q41 (rs1159268, P combined =4.08 × 10 −8 , OR=1.17). All three loci contain genes linked to the TGFβ cell signalling pathway, namely OVOL1 , FST and TGFB2 . Transcripts of OVOL1 and TFGB2 have decreased expression in affected compared with normal skin. Collectively, these data support a key role for dysregulation of TGFβ-mediated signalling in susceptibility to acne. A cne vulgaris (acne) is a chronic, inflammatory skin disease characterized by papules, pustules and nodules arising on the face, chest and back. These clinical features reflect underlying sebaceous gland hyperactivity, overgrowth of Propionibacterium acnes and inflammation of hair follicles [1] . Typically, the onset of acne occurs during puberty and may persist for many years with irreversible scarring occurring in up to 20% of patients. The consequent social and economic burden is profound with elevated rates of unemployment, depression and low self-esteem [1] , [2] in those affected. Family and twin studies indicate a substantial genetic contribution to acne susceptibility with heritability estimates of 78 and 81% (refs 1 , 3 ). Genome-wide association studies (GWAS) have made a substantial contribution to the understanding of the genetic basis of several common cutaneous inflammatory disorders [4] , [5] . However, efforts to characterize the genetic basis of acne have thus far been limited [6] , [7] . In the Han Chinese population, two genome-wide significant acne susceptibility loci (1q24.2 and 11p11.2) have recently been identified through the study of 1,056 acne cases and 1,056 controls [6] . The modest effect size (odds ratio (OR) of 1.22 and 1.23, respectively) of the reported loci together with the high heritability of acne suggest that additional well-powered GWAS, including studies in different populations, will provide an opportunity to discover further genetic determinants. Here we capitalized on a national network of dermatologists within the United Kingdom [8] to recruit subjects with severe acne and perform a case–control GWAS leading to the discovery of three new genome-wide significant association signals for acne. DNA from 2,001 individuals with severe acne was genotyped on the Illumina HumanOmniExpress-12v1_H microarray and compared with genotypes from 5,139 UK control subjects previously assayed [9] on the Illumina custom Human1.2M-Duo array. Association analysis was performed with 7.3 million variants that were imputed from the 1000 Genomes Phase I integrated variant set (April 2012) [10] based on genotypes at 386,674 single-nucleotide polymorphisms (SNPs) that had been successfully genotyped in cases and controls. Following quality control and imputation, high-quality data were available for 1,893 cases and 5,132 controls. We performed single SNP analysis using score tests under a logistic regression model including the first four principal components ( Supplementary Fig. 1a,b ) as covariates. The quantile–quantile plot indicated adequate control for confounders ( λ GC =1.037; Supplementary Fig. 1c ). We found no evidence for association at the acne risk loci reported in the Han Chinese population (1q24.2 (rs7531806, P discovery =0.597) and 11p11.2 (rs747650, P discovery =0.337; and rs1060573, P discovery =0.313)). Despite the absence of association at the two reported acne loci, examination of the quantile–quantile plot revealed a modest deviation from the null distribution, indicating an excess signal of association. We therefore selected 350 SNPs with evidence of association (Methods section; Supplementary Fig. 1d ) in the discovery cohort for a second-stage study. 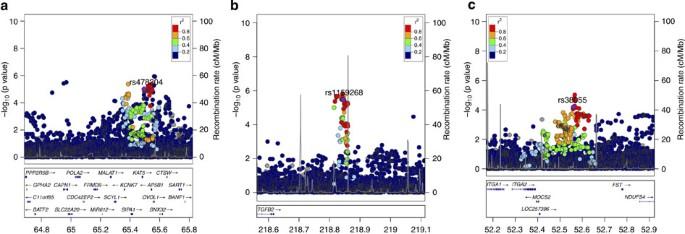Figure 1: Regional association plots at the three genome-wide significant loci. (a) 11q13.1, (b) 1q41 and (c) 5q11.2. The −log10Pdiscoveryvalues for the SNPs are shown on the leftyaxis of each plot. SNPs are coloured based on theirr2with the labelled lead SNP.r2is calculated from the 1000 Genomes (March 2012) genotypes. The bottom section of each plot shows the fine-scale recombination rates (rightyaxis) estimated from individuals in the 1000 Genomes population, and genes are marked by horizontal blue lines. Thexaxis shows the chromosomal position in Mb. We recruited a further 2,207 UK subjects with acne and performed a comparison with 2,087 controls from the Twins UK registry with self-reported absence of a history of acne [3] (Methods section; Supplementary Methods and Supplementary Table 1 ). Following quality control, high-quality genotypes were available for 286 SNPs across 2,063 cases and 1,970 controls. The second-stage analysis identified 13 SNPs surpassing nominal significance for association ( P second stage <0.05) with the same risk allele as identified in the discovery stage of this study. Of these, five SNPs achieved genome-wide significance in a meta-analysis of the discovery and second-stage cohorts ( P combined <5 × 10 −8 ; Table 1 and Fig. 1a–c ). Three of these SNPs are located within close proximity at 11q13.1 ( Fig. 1a ). Analysis conditioning on the lead SNP in this region (rs478304, P combined =3.23 × 10 −11 , OR=1.20) reduces the signal at the other two SNPs (rs610037 and rs72922786) to background, implying that a single signal underlies the observed association at these three SNPs. Two further genome-wide significant associations were identified at 5q11.2 (rs38055, P combined =4.58 × 10 −9 , OR=1.17) and 1q41 (rs1159268: P combined =4.08 × 10 −8 , OR=1.17). We found no evidence for interaction between SNPs at these three loci. Table 1 Loci showing genome-wide significant association with acne. Full size table Figure 1: Regional association plots at the three genome-wide significant loci. ( a ) 11q13.1, ( b ) 1q41 and ( c ) 5q11.2. The −log 10 P discovery values for the SNPs are shown on the left y axis of each plot. SNPs are coloured based on their r 2 with the labelled lead SNP. r 2 is calculated from the 1000 Genomes (March 2012) genotypes. The bottom section of each plot shows the fine-scale recombination rates (right y axis) estimated from individuals in the 1000 Genomes population, and genes are marked by horizontal blue lines. The x axis shows the chromosomal position in Mb. Full size image We considered genes located within 500 kb of each of the three lead SNPs as potential candidates for a role in acne pathogenesis [5] . In total, these three segments harbour 58 transcripts of which 39 are expressed in skin [11] . TGFB2 is the closest gene to the association signal at 1q41, located 226 kb from the lead SNP rs1159268. TGFB2 is a member of the transforming growth factor-β (TGFB) family of cytokines, and we noted that genes encoding proteins linked to the TGFβ cell signalling pathway are located within the regions of association at the other two genome-wide significant loci, namely OVOL1 (refs 12 , 13 , 14 ) at 11q13.1 and FST [15] at 5q11.2. The observation that a gene related to the TGFβ pathway is located in each of the three genome-wide significant loci identified in the current study is highly significant ( P =6 × 10 −5 , Methods section). We confirmed the presence of TGFB2, OVOL1 and FST transcripts in skin biopsies from individuals with acne and noted a significant reduction in TGFB2 ( P adjusted =6 × 10 −4 ) and OVOL1 ( P adjusted =4 × 10 −2 ) transcript levels in lesional compared with non-lesional skin ( Fig. 2a–c ). 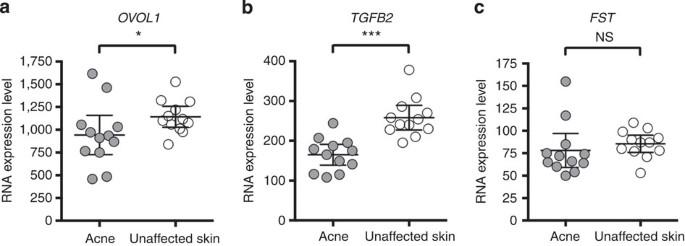Figure 2: Expression of associated genes in acne. Normalized expression of associated probe sets for respective genes on Affymetrix RNA expression chips (229396_atOVOL1, 228121_atTGFB2and 207345_atFST) in 12 biopsies of inflammatory acne papules compared with uninvolved skin of the same patients, samples plotted as circles and the overall mean is shown with the 95% confidence interval. Twenty-one of total 39 detected gene transcripts in skin are differentially expressed between lesional and non-lesional skin (Methods section). Stars indicate level of significance of pairedt-test after Benjamini–Hochberg correction for 38,014 tests, FDR 0.05 (*P<0.05, ***P<0.001). NS, not significant. Figure 2: Expression of associated genes in acne. Normalized expression of associated probe sets for respective genes on Affymetrix RNA expression chips (229396_at OVOL1 , 228121_at TGFB2 and 207345_at FST ) in 12 biopsies of inflammatory acne papules compared with uninvolved skin of the same patients, samples plotted as circles and the overall mean is shown with the 95% confidence interval. Twenty-one of total 39 detected gene transcripts in skin are differentially expressed between lesional and non-lesional skin (Methods section). Stars indicate level of significance of paired t -test after Benjamini–Hochberg correction for 38,014 tests, FDR 0.05 (* P <0.05, *** P <0.001). NS, not significant. Full size image We report three genome-wide significant associated loci with severe acne, each of which contains a gene whose protein product is linked both to the TGFβ pathway and to skin homeostasis, ranging from keratinocyte proliferation to wound healing [16] , [17] , [18] . The biology of TGFβ is consistent with a role in acne pathogenesis. Keratinocyte hyperproliferation, which may lead to follicular obstruction and comedo formation in acne [19] , [20] , is inhibited by TGFβ [21] , [22] . Likewise, TGFβ decreases sebaceous gland lipid production [23] which is increased and altered in acne [24] , [25] . Finally, innate immune responses, elicited during microbial colonization by P. acnes [26] , [27] , may be modulated by TGFβ [28] . Accordingly, transcript levels of TGFB2 were significantly reduced in fresh inflammatory acne papules in comparison with normal skin ( Fig. 2b ), as were transcripts of OVOL1 ( Fig. 2a ). OVOL1 is expressed in human [29] and murine [16] skin, in both hair follicles and interfollicular epidermis [16] . It encodes a zinc-finger transcription factor that is a downstream target of TGFβ/BMP7–Smad4 signalling, a pathway known to regulate growth of keratinocytes [12] . TGFβ results in growth arrest of wild-type but not OVOL1 −/− keratinocytes [16] , [30] , and OVOL1 −/− mice have a thicker epidermis due to hyperproliferation of keratinocytes [16] . A putative role of OVOL1 in skin pathology is not limited to acne since an association signal at this locus has also been reported in atopic dermatitis [31] . The SNP (rs479844) associated with atopic dermatitis shows no evidence for association with acne in the current study ( P discovery =0.301) nor is it in linkage disequilibrium (LD) with the lead SNP (rs478304) of the acne association signal ( r 2 =0.17), suggesting that the association signals are distinct. Our third genome-wide association signal is at 5q11.2 close to the FST gene. Its soluble protein product follistatin binds and neutralizes members of the TGFβ superfamily [15] , including activin, which is involved in scar formation in skin. Accordingly, mice overexpressing follistatin display reduced wound healing [18] , whereas overexpression of activin results in epidermal thickening and dermal fibrosis in normal skin and enhanced granulation tissue formation after wounding [32] . Our study in European subjects did not detect associations at either of the two previously described acne risk loci [6] . We recognize that our study design, which used an unselected population control cohort in the discovery phase, may impact on the ability to detect true associations. However, the size of the discovery cohort provides sufficient power to detect risk loci with effect sizes of the magnitude reported in the Han Chinese ( Supplementary Fig. 2 ). The disparity may reflect differences in the population-specific genetic determinants [33] and the case and control recruitment criteria of the respective studies. Of interest, the identification of SELL , encoding the leukocyte migration protein selectin L [34] , as a candidate gene at one of the loci identified in the Han Chinese population highlights potential inflammatory mechanisms, while the candidate genes reported here relate to tissue remodelling processes. Both systems are thought to be critical in acne pathophysiology [25] , [35] . In summary, we report genome-wide significant associations at three independent genomic loci. This brings the total confirmed regions across the genome known to confer risk for acne to five. Although additional genetic and functional studies are required to clarify the causative alleles at each of the loci, our data support a role of the TGFβ pathway in predisposition to acne. The current small number of modest effect risk loci taken in the context of the high heritability for acne provides a strong motivation for further genetic analysis, including a search for rare variants, to further our understanding of predisposition to this important disorder. Clinical samples for genetic study The study was designed in accordance with the Declarations of Helsinki, and ethical approval was obtained from the NRES Committee London-Westminster (reference CLRN 05/Q0702/114). 17 UK clinical centres recruited and obtained informed consent from individuals with acne for the discovery stage study, and 39 UK centres for the second-stage study. Clinical assessment was undertaken by trained dermatologists using one or more of the following criteria for a diagnosis of severe acne: (a) nodulocystic disease; (b) ≥5 points in any body region assessed by the validated Leeds clinical acne score that uses a colour photographic acne grading scheme to evaluate the severity of involvement of body regions (face 0–12, chest 0–8 and back 0–8) [36] ; (c) requiring treatment with isotretinoin; and (d) presence of rare and severe forms of acne such as, for example, acne fulminans . Inclusion and exclusion criteria are detailed in the Supplementary Methods , and were the same for the discovery and second-stage cohorts that comprised 2,001 and 2,207 individuals with severe acne, respectively. DNA for the case cohorts was extracted from saliva samples collected with Oragene kits ( n =3,541) or from whole blood ( n =667). The controls for the discovery-stage cohort comprised 2,478 healthy blood donors from the United Kingdom Blood Service (UKBS) collection and 2,661 individuals from the 1958 Birth Cohort (58C) data set [9] ( http://www.wtccc.org.uk/ccc2/ ). In the second-stage study, 2,087 controls were selected from the Twins UK registry and were enriched (87%) for individuals with no history of acne based on self-completed questionnaire. Clinical samples for expression study Paired skin biopsies of lesional and non-lesional skin were obtained from the upper back of acne patients of European origin (11 males and 1 female). The mean age of patients was 23.5 years (± 3.6 years s.d.). All were untreated and had inflammatory acne with evidence of scarring. Acute inflammatory papules, defined as having developed within 48 h, were biopsied. Genotyping and quality control in discovery stage Genome-wide genotyping for the discovery case cohort was conducted by Illumina Corp. (CA) on Illumina HumanOmniExpress-12v1_H microarrays. Bead intensity data were processed and normalized for each sample in BeadStudio, data for successfully genotyped samples were extracted and genotypes were called using Illuminus (Illumina Corp.). Controls for the discovery stage had been previously genotyped on an Illumina 1.2M platform at the Sanger Institute, Cambridge [9] . Non-overlapping SNPs (255,193) that were only assessed in either cases or controls were excluded during merging of case and control data sets. Using the Plink software package, we followed accepted quality control procedures [37] and excluded 108 cases and 7 controls based on the following criteria: >2% missing genotypes, discrepancy of inferred gender with sample information, cryptic relatedness (PI_HAT>0.2, one of each pair of related individuals were excluded) and excessive heterozygosity. Population stratification was assessed using Principal Component Analysis (PCA) implemented in EIGENSOFT4.2 (refs 38 , 39 ) using an LD pruned ( r 2 <0.2) set of 93,906 autosomal SNPs that are not located within regions of long-range-LD [40] . Plots of PCA axis 1 and 2 identified 83 outlier samples (63 cases and 20 controls) who were excluded from further analysis and PCA was repeated. SNPs with a call rate <99%, Hardy–Weinberg equilibrium test P <10 −6 , MAF <0.5% or significantly different call rates between cases and controls ( P <0.05), and sex-chromosomal SNPs were removed from further analysis. After quality control, genotypes for 386,674 SNPs in 1,893 cases and 5,132 controls remained. Imputation and association testing in discovery stage Imputation was performed in a two-stage approach. Initially, the data were phased with ShapeIt [41] ( http://www.shapeit.fr ) and subsequently imputed against the 1000 Genomes reference panel [10] with IMPUTE2 (ref. 42 ; http://mathgen.stats.ox.ac.uk/impute/impute_v2.html ). SNPs imputed with relatively high confidence (estimated r 2 between imputed and true genotypes>0.5) were included in the analysis. SNPTEST v2.4.0 (ref. 43 ); ( https://mathgen.stats.ox.ac.uk/genetics_software/snptest/snptest.html ) was used for association testing using the first four covariates ( Supplementary Fig. 1a,b ) to correct for population stratification and other potential confounders. The over dispersion factor of association test statistics λ was 1.037, suggesting that the impact of systematic differences between cases and controls were within acceptable limits ( Supplementary Fig. 1c,d ). SNP selection for second-stage study In total, 350 SNPs were selected for the second-stage study ( Supplementary Data 1 ), 108 lead SNPs with a P discovery <1 × 10 −5 that represent the strongest evidence of statistical association at each respective locus. A further 242 SNPs with a P discovery <1.3 × 10 −3 were selected as either proxies for the lead SNPs or located in close proximity to genes highly expressed in skin ( SDC1 and TYRP1 ), published candidate genes ( CYP21A2 (ref. 44 ) or other putative roles in tissue remodelling ( FGF2 and FGF22 ) or the immune response ( IL1R1/2, IL1RL1/2, IL18R1, ICAM4 and CFB ). We preferentially selected genotyped over imputed SNPs and SNPs with a minor allele frequency of >0.02, including manual inspection of cluster plots of genotyped SNPs. Genotyping, quality control and association testing in second stage Genotyping was undertaken at the KCL/GSTT BRC Genomics Core Facility using the Illumina GoldenGate assay (GT-221-1109-GGGT Universal-32). The generated data were subject to sample and SNP quality control procedures as described above, including visual inspection of cluster plots. We fitted a logistic regression model for case or control status with no covariates at each SNP and a single parameter for the genetic effect (a multiplicative effect on the risk scale and an additive effect on the log-odds scale). The inflation was λ =1.047. Of the 350 SNPs selected for the second stage, 286 passed quality control and genotypes were available for 2,063 cases and 1,970 controls ( Supplementary Data 1 ). Of these, 18 achieved nominal significance ( P second stage <0.05) of which 13 (4.5%) were directionally consistent with the same risk allele as was observed in the discovery study. Seven of the 108 second-stage SNPs passing quality control and whose selection was based solely on statistical criteria ( P discovery <10 −5 ) achieved nominal significance (six directionally consistent with the discovery study). The controls of the second-stage study were predominantly female ( Supplementary Table 1 ). As our analyses were limited to autosomal regions of the genome, Mendelian segregation ensures that the analysed genotypes and gender are uncorrelated. We tested to establish whether the genetic effects were modulated by gender (modelling SNP allele dosage+gender+gender × dosage+the first four principal components as covariates), which failed to demonstrate an interaction for any of the genome-wide significant SNPs ( P -values for interaction term: rs38055, P =0.57; rs478304, P =0.22; and rs1159268 P =0.99). Researchers can request access to the data via email to the corresponding authors or via the relevant data access committee ( http://www.ebi.ac.uk/ega ; http://www.twinsuk.ac.uk/data-access/ ). Regional plots and identification of genes within associated regions Associated regions were plotted using the stand-alone version of LocusZoom [45] using the P discovery values from the discovery study and LD information from the 1000 Genomes Project. Regions of association were defined by a 500-kb interval flanking each association signal [5] . Evaluation of the observation of TGFβ-associated genes within the genome-wide association signals Overlapping 500 kb regions flanking the SNPs passing quality control in the second stage were merged, resulting in 180 distinct loci of 1.06 Mb on average (s.d. 0.3 Mb). The genes in the 177 loci interrogated in the second stage in which we did not observe genome-wide signals were mapped to the Kyoto Encyclopedia of Genes and Genomes (KEGG) TGFβ pathway, identifying five genes ( MYC, SMAD1, TNF, MAPK3 and GDF7). A hypergeometric exact test [46] was used to evaluate the probability of the observation of three genes linked to the TGFβ pathway located in three genome-wide significant loci when a total of eight such genes are present across all 180 loci. Conditional analysis We observed three SNPs (rs478304, rs610037 and rs72922786) with genome-wide significance at the 11q13.1 locus. We performed conditional analysis on the second-stage data set, conditioning the analysis of rs610037 and rs72922786 with the observed genotypes of the lead SNP rs478304. Skin expression studies Punch biopsies were immediately transferred to RNAlater Tissue Protect Tubes (Qiagen). Total RNA was extracted using miRNeasy extraction kits (Qiagen) including DNase I treatment (27U, 15 min). All RNA samples were evaluated by NanoDrop 8800 and displayed a good profile with a RNA Integrity Number >7 and a concentration >60 ng μl −1 . cRNA labelling and hybridization were performed according to Affymetrix protocols. Biotinylated RNA and fragmented RNA were assessed for relative length on an Agilent 2100 bioanalyzer. Fragmented RNA was hybridized on Affymetrix U133 Plus 2.0 chips. Affymetrix RMA (Robust Multichip Average) software was used to perform the quality control of the study before analysing the data, namely normalized using the RMA method. RMA consists of three steps: background adjustment, quantile normalization and finally summarization. Genes within a 500-kb interval (see above) of the association signals were assessed for transcript abundance and differential expression between lesional and non-lesional skin. Statistical analysis was performed with paired two-tailed t -test adjusted for 38,014 independent tests. How to cite this article: Navarini, A.A. et al. Genome-wide association study identifies three novel susceptibility loci for severe Acne vulgaris . Nat. Commun. 5:4020 doi: 10.1038/ncomms5020 (2014).